A disinhibitory mechanism biasesDrosophilainnate light preference 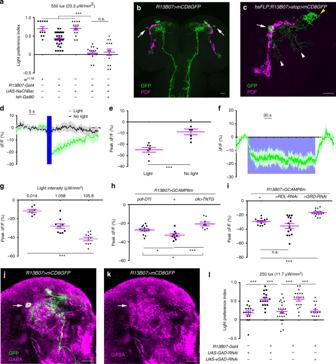Fig. 1 Light inhibition of GABAergic LRINR13B07s in brain is required for larval light avoidance.aActivation ofR13B07-Gal4neurons in brain abolishes larval avoidance to white light at 550 lux (23.3 μW/mm2).bExpression pattern ofR13B07-Gal4in larval brain. Arrows point to the LRINR13B07s.cMorphology of single LRINR13B07. Arrow, yellow and white arrow heads, respectively, point to the cell body, axonal termini and dendrites of LRINR13B07.d–eLRINR13B07s are inhibited by 470 nm light at intensity of 1.058 μW/mm2.eis the statistics of the peak calcium responses ind.fSustained inhibition on LRINR13B07s by light. 470 nm light at intensity of 0.001 μW/mm2was used.n= 3.gExtent of inhibition on LRINR13B07s is increased as light intensity increases. 470 nm light at intensity of 0.014 μW/mm2, 1.058 μW/mm2, and 105.8 μW/mm2was used for 3 s.hBlockingclk-LexAlabeled neurons or knocking outpdfneurons reduces the inhibition of LRINR13B07s by light. 470 nm light at intensity of 105.8 μW/mm2was used for 3 s. The genotypes ofpdf-DTI/UAS-GCAMP6m;R13B07-Gal4/+,UAS-GCAMP6m/+;R13B07-Gal4/+andclk-LexA/UAS-GCAMP6m;R13B07-Gal4/ LexAop-TNTGare used.iKnocking down GRD expression in LRINR13B07s reduced the inhibition of LRINR13B07s by light. 470 nm light at intensity of 1.058 μW/mm2was used for 3 s. The genotypes areUAS-GCAMP6m/+;R13B07-Gal4/+,UAS-GCAMP6m/UAS-RDL-RNAi;R13B07-Gal4/+andUAS-GCAMP6m/UAS-GRD-RNAi;R13B07-Gal4/+, respectively.j–kSingle slice view of anti-GABA staining against LRINR13B07. Arrows point to the co-localization in cell body of LRINR13B07.jis the channel for GABA ini.lKnocking down expression of GAD or vGAT in LRINR13B07s enhances larval avoidance to white light at 250 lux (11.7 μW/mm2). The blue bars indand violet block infindicate periods of light stimulation. Scale bars, 20 μm inb–candj–k. n.s. not significant, *P< 0.05, **P< 0.01, ***P< 0.001,t-test ine, one-way ANOVA ing, one-way ANOVA with Tukey’s post hoc test ina,h,i, andl. Error bars, SEMs. Source data ofa,d–i,lare provided as a source data file Innate preference toward environmental conditions is crucial for animal survival. Although much is known about the neural processing of sensory information, how the aversive or attractive sensory stimulus is transformed through central brain neurons into avoidance or approaching behavior is largely unclear. Here we show that Drosophila larval light preference behavior is regulated by a disinhibitory mechanism. In the disinhibitory circuit, a pair of GABAergic neurons exerts tonic inhibition on one pair of contralateral projecting neurons that control larval reorientation behavior. When a larva enters the light area, the reorientation-controlling neurons are disinhibited to allow reorientation to occur as the upstream inhibitory neurons are repressed by light. When the larva exits the light area, the inhibition on the downstream neurons is restored to repress further reorientation and thus prevents the larva from re-entering the light area. We suggest that disinhibition may serve as a common neural mechanism for animal innate preference behavior. When choosing between two alternative conditions, animals such as Drosophila larva reorientates when facing unfavorable conditions but maintain unchanged directions when facing favorable conditions [1] , [2] , [3] . The choice behavior involves transforming sensory input into motor action of reorientation. In vertebrates, although the brain regions or neurons that are responsible for sensory information processing and motor control have been relatively well mapped [4] , [5] , the cellular and molecular mechanism underlying sensorimotor transformation in central brain has only been reported in a few cases, such as cutaneous or olfactory input-induced locomotion in xenopus and lamprey [6] . In Drosophila larva, Bolwig’s organs, i.e. the photoreceptors, regulate larval avoidance response to light in both laboratory and outdoor experiments [7] , [8] , [9] , [10] , [11] , [12] . Bolwig’s organs directly send projections into the larval optical neuropil (LON) in central brain and synapse on visual local neurons and visual projection neurons [13] . These downstream neurons, including visual local neurons such as lOLP (local optic lobe pioneer) neurons, and visual projection neurons such as pdf neurons and 5 th lateral neuron in clock circuit as well as PVL09 neurons (posterior-ventro-lateral neuron 09), have been reported to be involved in various forms of larval light navigational behaviors [7] , [9] , [11] , [12] , [14] . At the level of motor control, neurons in Drosophila larval SEZ (subesophageal zone) have been suggested to command larval reorientation behavior in light avoidance [15] . But the neuronal circuitry that bridges the gap between upstream visual processing neurons and downstream turning command neurons has been left blank [16] . How the visual signal is transformed into an avoidance behavior remains largely elusive. Disinhibition is a central mechanism that serves in various neural functions, such as sensory signal processing [17] , [18] , [19] , selection of motor programs [20] , [21] , memory expression [22] , and the switch between wake and sleep status [23] . In a disinhibitory microcircuit, the inhibition on downstream inhibitory neurons is supposed to be tonic, whereas the inhibition on upstream inhibitory neurons should be phasic [20] , [24] , [25] . This enables the efficient temporal control of the excitability of the downstream neurons. Here we show that Drosophila larval avoidance to light is gated in a disinhibitory manner. We propose that disinhibition is the underlying mechanism for the initiation of choice action and subsequent securement of the correct choice in animal choice behavior. Larval light avoidance requires inhibition of LRIN R13B07 s To discover neurons that inhibit Drosophila larval reorientation in light avoidance, we crossed Gal4 lines with UAS-NaChBac which increases neuronal excitability and tested the larvae in a light/dark choice assay at a light intensity of 550 lux (23.3 μW/mm 2 ). 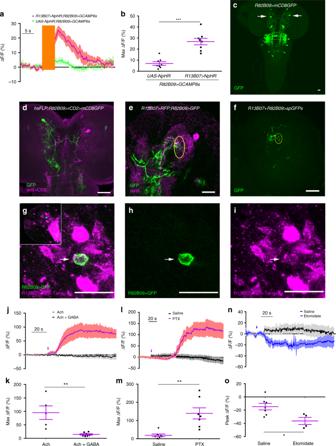Fig. 2 RDL on CLPNR82B09s mediates the inhibition from LRINR13B07sa–b. Optogenetic inhibition of LRINR13B07s allows excitation of CLPNR82B09s.bis the statistics of peak calcium responses ina. The orange bar indicates the 540 nm light stimulation. The genotypes areR82B09-LexA/UAS-NpHR; LexAop-GCAMP6s/+andR82B09-LexA/UAS-NpHR; R13B07-Gal4/ LexAop-GCAMP6s.cExpression pattern ofR82B09-Gal4in larval brain. Arrows point to cell bodies of CLPNR82B09s.dMorphology of single CLPNR82B09labeled byR82B09-Gal4.eCo-localization between the dendrites of CLPNR82B09and LRINR13B07in larval brain. Yellow circle outlines the overlapping region between LRINR13B07and CLPNR82B09.fGRASP signal between CLPNR82B09and LRINR13B07. Yellow circle outlines verified contact region.g–itrans-Tango probes CLPNR82B09as immediate downstream ofR13B07-Gal4labeled neuron.gis the merged version ofhandi. trans-Tango signal is in magenta. GFP signal driven byR82B09-Gal4is in green. Arrows indicated the overlapping between trans-Tango signal and GFP signal that labels the cell body of a CLPNR82B09. Inset ingshows the position of the co-localization in larval brain hemisphere.UAS-myrGFP,QUAS-mtdTomato(3xHA)/+;trans-Tango/+;R13B07-Gal4/R82B09-Gal4is the genotype of the larva used. trans-Tango signals are reported by 3xHA.j–kApplication of 100 mM GABA repressed the activation of CLPNR82B09s by 100 μM acetycholine.his the statistics of peak calcium responses ing.l–mApplication of 100 μM RDL antagonist picrotoxin allows excitation of CLPNR82B09s.jis the statistics of peak calcium responses ini.n–oCalcium response in CLPNR82B09s before and after etomidate application. Arrow indicates application of drug.ois the statistics of peak responses inn. Scale bars, 20 μm inc–i. Samples inj–owere prepared from larvae of genotypeR82B09-LexA;LexAop-GCAMP6s. Arrows indicate application of drugs inj,l, andn. *P< 0.05, **P< 0.01, ***P< 0.001,t-test inb,k,m, ando. Error bars, SEMs. Source data ofa–bandj–oare provided as a source data file One Gal4 line of R13B07-Gal4 that labeled about seven to ten interneurons in the anterior part of each larval brain hemisphere and a group of neurons in posterior part of VNC (ventral nerve cord), in addition to the Rh6-positive photoreceptors in peripheral nervous system, demonstrated an abolished larval light avoidance (Fig. 1a, b , Supplementary Fig. 1 , Supplementary Fig. 2 a–c). This defect was not rescued by introduction of tsh-Gal80 that specifically represses Gal4 activity in VNC, suggesting that larval light avoidance did not involve the R13B07-Gal4 labeled neurons in the VNC (Fig. 1a , Supplementary Fig. 1 a–c). As hyperactivating Rh6-positive neurons alone did not affect larval light avoidance, they could also be excluded (Supplementary Fig. 2d ). So it should be the neurons in brain hemispheres that repressed larval light avoidance. Fig. 1 Light inhibition of GABAergic LRINR13B07s in brain is required for larval light avoidance. a Activation of R13B07-Gal4 neurons in brain abolishes larval avoidance to white light at 550 lux (23.3 μW/mm 2 ). b Expression pattern of R13B07-Gal4 in larval brain. Arrows point to the LRIN R13B07 s. c Morphology of single LRIN R13B07 . Arrow, yellow and white arrow heads, respectively, point to the cell body, axonal termini and dendrites of LRIN R13B07 . d – e LRIN R13B07 s are inhibited by 470 nm light at intensity of 1.058 μW/mm 2 . e is the statistics of the peak calcium responses in d . f Sustained inhibition on LRIN R13B07 s by light. 470 nm light at intensity of 0.001 μW/mm 2 was used. n = 3. g Extent of inhibition on LRIN R13B07 s is increased as light intensity increases. 470 nm light at intensity of 0.014 μW/mm 2 , 1.058 μW/mm 2 , and 105.8 μW/mm 2 was used for 3 s. h Blocking clk-LexA labeled neurons or knocking out pdf neurons reduces the inhibition of LRIN R13B07 s by light. 470 nm light at intensity of 105.8 μW/mm 2 was used for 3 s. The genotypes of pdf-DTI/UAS-GCAMP6m;R13B07-Gal4/ + , UAS-GCAMP6m/ + ; R13B07-Gal4/ + and clk-LexA/UAS-GCAMP6m;R13B07-Gal4/ LexAop-TNTG are used. i Knocking down GRD expression in LRIN R13B07 s reduced the inhibition of LRIN R13B07 s by light. 470 nm light at intensity of 1.058 μW/mm 2 was used for 3 s. The genotypes are UAS-GCAMP6m / + ; R13B07-Gal4 / + , UAS-GCAMP6m/UAS-RDL-RNAi;R13B07-Gal4/ + and UAS-GCAMP6m/UAS-GRD-RNAi;R13B07-Gal4/ + , respectively. j – k Single slice view of anti-GABA staining against LRIN R13B07 . Arrows point to the co-localization in cell body of LRIN R13B07 . j is the channel for GABA in i . l Knocking down expression of GAD or vGAT in LRIN R13B07 s enhances larval avoidance to white light at 250 lux (11.7 μW/mm 2 ). The blue bars in d and violet block in f indicate periods of light stimulation. Scale bars, 20 μm in b – c and j – k . n.s. not significant, * P < 0.05, ** P < 0.01, *** P < 0.001, t -test in e , one-way ANOVA in g , one-way ANOVA with Tukey’s post hoc test in a , h , i , and l . Error bars, SEMs. Source data of a , d – i , l are provided as a source data file Full size image As activation of these neurons negatively regulated light avoidance, we hypothesized that these neurons might be inhibited by light. We then tested the responses of the brain hemisphere neurons to light in calcium imaging. Among these neurons, only one pair of anterio-laterally localized neurons that each possessed a comprehensive dendritic region posterior-medial to the cell body and a dense sytGFP labeled axonal arborization region anterio-medial to the dendrites (Fig. 1c , Supplementary Fig. 1 e, f), was strongly inhibited by blue light stimulation (Fig. 1d, e ). As these neurons turned out to be inhibitory later, we named these R13B07-Gal4 labeled light repressed inhibitory neurons LRIN R13B07 s. The inhibition persisted as light was on for up to 3 min (Fig. 1f ). When light intensity increased, this inhibition was strengthened (Fig. 1g ). As the dendritic regions of the neurons were adjacent to the axonal projection area of lateral clock neurons outlined by anti-PDF, we reasoned that they might receive visual inputs from the clock neurons (Fig. 1c ) [12] , [14] , [26] . We made use of a R43D05-LexA line that was generated using a fragment of the promoter of clock(clk) gene. This line labeled pdf neurons and neurons that were morphologically similar to the fifth lateral neurons (5 th LN), DN1 (dorsal neuron 1), DN2 (dorsal neuron 2), in addition to three clusters of putatively immature neurons in each brain hemisphere (Supplementary Fig. 3 ). When the clk-LexA labeled neurons were blocked with TNTG, a presynaptic inhibitor of neurotransmission, the extent of the inhibition was significantly reduced, suggesting that the inhibition at least partially originated from the clk-LexA labeled neurons (Fig. 1h ). Specifically ablating pdf neurons using pdf-DTI (DTI, diphtheria toxin) could also relieve the light-induced inhibition, but obviously not as effective as inhibiting clk-LexA neurons (Fig. 1h ). We next asked which receptor was used by LRIN R13B07 s to receive the inhibitory input. Knocking down in LRIN R13B07 s the expression of a GABA/Glycine receptor GRD [27] , [28] , but not of another GABA receptor RDL [29] , could efficiently reduce the extent of inhibition (Fig. 1i ). This meant that the inhibition of LRIN R13B07 s by light was mediated by the GRD receptor. LRIN R13B07 s are GABAergic As the LRIN R13B07 s were inhibited by light and the activation of LRIN R13B07 s suppressed larval light avoidance, we reasoned that these light inhibited neurons might inhibit other neurons that promote light avoidance. We co-stained the antibody against GABA, the most widely used inhibitory neurotransmitter, with R13B07-Gal4 to test whether they were indeed inhibitory. The anti-GABA signal indeed co-localized well with the cell bodies of the LRIN R13B07 s (Fig. 1j, k ). LRIN R13B07 s signal did not co-localize with anti-ChAT (choline acetyltransferase) that marks the cholinergic neurons, but about three other R13B07-Gal4 labeled neurons in each larval brain hemisphere did (Supplementary Fig. 1 g–i). This was verified by our observation that introduction of Cha-Gal80 reduced the number of R13B07-Gal4 labeled neurons by about three in each brain hemisphere (Supplementary Fig. 1j ). The remaining labeling of axonal termini of photoreceptor neurons might be due to insufficient repression on Gal4 activity by Cha-Gal80 . On the other hand, vGlut-Gal80 , which was assumed to be expressed in glutamatergic neurons, did not obviously affect the expression of R13B07-Gal4 in larval brain (Supplementary Fig. 1k ). We then tested the role of GABA in LRIN R13B07 s in larval light avoidance using the light/dark choice assay. When we knocked down expression of GABA synthesizing enzyme GAD (glutamate decarboxylase) or vesicular GABA transporter vGAT (vesicular GABA transporter) in the LRIN R13B07 s, larval light avoidance was enhanced (Fig. 1l ). It should be noted that we used relatively weaker light of 250 lux (11.7 μW/mm 2 ) instead of 550 lux (23.3 μW/mm 2 ) in the assay to reduce the level of light avoidance in control lines, thus making more space for further improvement in light preference index. Although the possibility that LRIN R13B07 s were cholinergic or glutamatergic could not be completely excluded based on absence of labeling, they were the only R13B07-Gal4 labeled neurons that were GABAergic and inhibited by light. Therefore, they should be the neurons that were responsible for larval light avoidance among all the R13B07-Gal4 labeled neurons. As LRIN R13B07 s were inhibitory neurons that were inhibited by light, larval light avoidance thus might be regulated by a disinhibitory mechanism [18] , [19] , [20] , [21] , [22] , [23] . LRIN R13B07 s inhibit CLPN R82B09 s We next searched for the light avoidance promoting neurons downstream of LRIN R13B07 s. Inhibition of the LRIN R13B07 s using an optogenetic tool NpHR induced a robust calcium signal increase in one pair of central brain neurons labeled by R82B09-Gal4 (Fig. 2a–c ), suggesting that these neurons had been subjected to tonic inhibition from the LRIN R13B07 s. These contralateral projecting neurons were then named as CLPN R82B09 s. They were also labeled by R82B09-LexA and R82B10-Gal4 (Supplementary Fig. 4a-c ). The CLPN R82B09 had a small axonal arborization region in the medial contralateral brain hemisphere, a widespread dendritic region near the dendrites of the LRIN R13B07 s, and a smaller dendritic arborization area in larval SEZ (Fig. 2 d, Supplementary Fig. 4 d–f). The dendrites of LRIN R13B07 s were found to be overlapping with the dendrites of the CLPN R82B09 s (Fig. 2e ). We then used GRASP technique to confirm the contact between LRIN R13B07 s and CLPN R82B09 s. A strong GRASP signal was seen in the overlapping region (Fig. 2f , Supplementary Fig. 5 ). The putative synaptic contact was validated by trans-Tango [30] , a newly developed technique that can be used to probe downstream synaptic partners of neurons. By driving expression of trans-Tango with R13B07-Gal4 to search for immediately downstream neurons, a large amount of cells were successfully marked (Supplementary Fig. 6a–b ). Some of these cells were in the same region of CLPN R82B09 s (Supplementary Fig. 6b ). We then added R82B09-Gal4 in the system to see if the trans-Tango signals driven by R13B07-Gal4 overlap with the GFP signals that marked CLPN R82B09 . As expected, co-localization was readily found (Fig. 2g–i ). This result was in support of a direct dendrodendritic interaction between LRIN R13B07 s and CLPN R82B09 s, as driving trans-Tango using R82B09-Gal4 alone did not yield any CLPN R82B09 signal (Supplementary Fig. 6 c, d). As LRIN R13B07 s were GABAergic, we reasoned that CLPN R82B09 s should be subjected to direct GABAergic inhibition. Fig. 2 RDL on CLPN R82B09 s mediates the inhibition from LRIN R13B07 s a – b . Optogenetic inhibition of LRIN R13B07 s allows excitation of CLPN R82B09 s. b is the statistics of peak calcium responses in a . The orange bar indicates the 540 nm light stimulation. The genotypes are R82B09-LexA/UAS-NpHR; LexAop-GCAMP6s/ + and R82B09-LexA/UAS-NpHR; R13B07-Gal4/ LexAop-GCAMP6s . c Expression pattern of R82B09-Gal4 in larval brain. Arrows point to cell bodies of CLPN R82B09 s. d Morphology of single CLPN R82B09 labeled by R82B09-Gal4 . e Co-localization between the dendrites of CLPN R82B09 and LRIN R13B07 in larval brain. Yellow circle outlines the overlapping region between LRIN R13B07 and CLPN R82B09 . f GRASP signal between CLPN R82B09 and LRIN R13B07 . Yellow circle outlines verified contact region. g – i trans-Tango probes CLPN R82B09 as immediate downstream of R13B07-Gal4 labeled neuron. g is the merged version of h and i . trans-Tango signal is in magenta. GFP signal driven by R82B09-Gal4 is in green. Arrows indicated the overlapping between trans-Tango signal and GFP signal that labels the cell body of a CLPN R82B09 . Inset in g shows the position of the co-localization in larval brain hemisphere. UAS-myrGFP,QUAS-mtdTomato(3xHA)/ + ;trans-Tango/ + ;R13B07-Gal4/R82B09-Gal4 is the genotype of the larva used. trans-Tango signals are reported by 3xHA. j – k Application of 100 mM GABA repressed the activation of CLPN R82B09 s by 100 μM acetycholine. h is the statistics of peak calcium responses in g . l – m Application of 100 μM RDL antagonist picrotoxin allows excitation of CLPN R82B09 s. j is the statistics of peak calcium responses in i . n – o Calcium response in CLPN R82B09 s before and after etomidate application. Arrow indicates application of drug. o is the statistics of peak responses in n . Scale bars, 20 μm in c – i . Samples in j – o were prepared from larvae of genotype R82B09-LexA;LexAop-GCAMP6s . Arrows indicate application of drugs in j , l , and n . * P < 0.05, ** P < 0.01, *** P < 0.001, t -test in b , k , m , and o . Error bars, SEMs. Source data of a – b and j – o are provided as a source data file Full size image To confirm this hypothesis, we applied drugs to dissected and digested larval brain samples, in which CLPN R82B09 s were disassociated and more susceptible to drug application. GABA could efficiently repress the excitation of CLPN R82B09 s induced by acetycholine in calcium imaging (Fig. 2j, k ). This result meant that CLPN R82B09 s indeed subjected to GABAergic inhibition, in addition to cholinergic excitation. Furthermore, the application of RDL antagonist picrotoxin could strongly activate CLPN R82B09 s (Fig. 2l, m ), while RDL agonist etomidate could efficiently inhibit CLPN R82B09 s (Fig. 2n, o ). Together, these data suggested that CLPN R82B09 s used RDL to receive GABAergic inhibitory input from LRIN R13B07 s. Light responsive CLPN R82B09 s control larval reorientation We next examined if CLPN R82B09 s were required for larval light avoidance. Blocking CLPN R82B09 s by expression TNTG with either R82B09-Gal4 or R82B10-Gal4 abolished larval preference for darkness in the light/dark choice assay at 550 lux (23.3 μW/mm 2 ) (Fig. 3a ). Introduction of Cha-Gal80 which removed Gal4 activity in all neurons except CLPN R82B09 s did not rescue the defect (Fig. 3a and Supplementary Fig. 4c ). Additionally, knocking down RDL expression in CLPN R82B09 s enhanced the larval preference for darkness over light when a relatively weaker light intensity of 250 lux (11.7 μW/mm 2 ) was used (Fig. 3b ). On the other hand, when we expressed UAS-Chrimson with R82B10-Gal4 to activate the CLPN R82B09 s, robust larval head casts were observed (Fig. 3c, d ). This could even be realized by optogenetic activation of a single CLPN R82B09 (Supplementary Video 1 ). These results suggested that the CLPN R82B09 s might control light-induced head cast. Indeed, our calcium imaging results showed that the CLPN R82B09 s did respond to light stimulation (Fig. 3e, f ). It is noted that the calcium transient could last for up to 40 s, whereas larval light avoidance response generally takes only at most a few seconds. The long duration of calcium response was likely due to dissection of larval body before calcium imaging that greatly changed the physiological environment of the imaged neurons. Knocking down RDL expression in the CLPN R82B09 s not only increased the probability (see Methods for more details) (Fig. 3g ), but also significantly improved the amplitude of the response (Fig. 3e, f ). As a neuronal calcium transient usually reflects the accumulative effect of a bout of action potentials, the increased probability in calcium response reflected greater chance for burst of action potentials [31] , [32] , [33] . We further asked if the light input to CLPN R82B09 s was also mediated by the known visual pathway neurons such as the clk-LexA labeled neurons and pdf neurons. Inhibiting clk-LexA neurons using TNTG significantly reduced the probability but not the amplitude of CLPN R82B09 s’ light response in calcium imaging (Fig. 3h, i ). However, ablating pdf neurons using pdf-DTI affected neither the probability nor the amplitude (Supplementary Fig. 7 ). This meant that at least part of the light signal transmitted to CLPN R82B09 s was through the clk-LexA neurons and this part of signal might decide whether CLPN R82B09 s responded to light or not, but not how strong the responses were. The above results together suggested that CLPN R82B09 s controlled the light-induced head cast in light avoidance. Fig. 3 The CLPN R82B09 s control head cast response to light. a Inhibiting CLPN R82B09 s abolishes larval avoidance to white light at 550 lux (23.3 μW/mm 2 ). b Knocking down RDL expression in CLPN R82B09 s enhances larval avoidance to white light at 250 lux (11.7 μW/mm 2 ). c – d Optogenetic stimulation of CLPN R82B09 s evokes larval head cast. d is the statistics of head cast sizes in c . The pink bar indicates the period of optogenetic stimulation. e – g Knocking down RDL expression in CLPN R82B09 s increases both amplitude and probability of CLPN R82B09 s’ response to light in calcium imaging. The blue bar in e indicates 470 nm light stimulation at intensity of 10.58 μW/mm 2 . f is the statistics of peak responses in e . h – i Blocking clk-LexA neurons with TNTG does not affect the amplitude ( h ), but undermines the probability of CLPN R82B09 s’ response to light in calcium imaging ( i ). One second 470 nm light stimulation at intensity of 10.58 μW/mm 2 was used. In e – i, R82B09 > GCAMP6m is the short for UAS-GCAMP6m/ + ;R82B09-Gal4/ + . R82B09 > GCAMP6m + RDL-RNAi is the short for UAS-GCAMP6m/UAS-RDL-RNAi;R82B09-Gal4/ + . clk > TNTG;R82B09 > GCAMP6m is the short for clk-LexA/UAS-GCAMP6m; R82B09-Gal4/LexAop-TNTG . Numbers above columns in g and i indicate sample sizes. n.s. not significant, * P < 0.05, ** P < 0.01, *** P < 0.001, one-way ANOVA with Tukey’s post hoc test in a – b , d , and f , t -test in h , fisher’s exact test in g and i . Error bars, SEMs. Source data of a – i are provided as a source data file Full size image Disinhibition of CLPN R82B09 s facilitates larval head cast Despite that light inhibits LRIN R13B07 s and LRIN R13B07 s inhibit CLPN R82B09 s, it was still not clear if the light-induced larval reorientation was regulated by disinhibition of CLPN R82B09 s through inhibition of LRIN R13B07 s. To confirm this hypothesis, we first tested whether the CLPN R82B09 s’ response to light was regulated by the LRIN R13B07 s- CLPN R82B09 s inhibition. Knocking down GRD expression in LRIN R13B07 s to reduce the light-induced inhibition on LRIN R13B07 s could significantly reduce the probability for CLPN R82B09 s to respond to light, while the amplitude of the response seemed to be unaffected (Fig. 4a and Supplementary Fig. 8 ). On the other hand, when we knocked down GAD expression in LRIN R13B07 s to relieve the GABAergic inhibition on CLPN R82B09 s, the probability for CLPN R82B09 s to respond to light was significantly improved, although the amplitude of the response was also unaffected (Fig. 4a and Supplementary Fig. 8 ). These results were in consistence with the effects of blocking clk-LexA neurons as shown in Fig. 3f, g . It was probably because blockage of clk-LexA neurons reduced light inhibition on LRIN R13B07 s that CLPN R82B09 s were no longer efficiently disinhibited. In the case of ablating pdf neurons, light inhibition on LRIN R13B07 s was also reduced but not as much as blocking clk-LexA neurons, so that the inhibition of CLPN R82B09 s by LRIN R13B07 s could still be relieved. Taken together, these results suggested that CLPN R82B09 ’s response to light was indeed gated by inhibition of LRIN R13B07 s. Fig. 4 Larval reorientation at light-on is facilitated by disinhibition of CLPN R82B09 s. a Knocking down GRD and GAD expression in LRIN R13B07 s, respectively, reduces and increases the probability for CLPN R82B09 s to respond to light in calcium imaging. One second 470 nm light stimulation at intensity of 1.058 μW/mm 2 was used. Numbers above columns indicate sample sizes. Genotypes of larvae used are R82B09-LexA/UAS-GRD-RNAi;LexAop-GCAMP6s/R13B07-Gal4 , R82B09-LexA/ + ;LexAop-GCAMP6s/ + and R82B09-LexA/UAS-GAD-RNAi;LexAop-GCAMP6s/R13B07-Gal4 , respectively. b – d Size of larval head cast at light-on in the light spot assay is reduced by downregulation of GRD in LRIN R13B07 s ( b ), but is enhanced by down regulation of GAD/vGAT in LRIN R13B07 s ( c) or RDL in CLPN R82B09 s ( d ). Light intensity in spot measured at 470 nm was 26.34 pW/mm 2 for b , 1.80 pW/mm 2 for c – d . * P < 0.05, ** P < 0.01, *** P < 0.001, χ 2 -test with subgroup comparisons controlled by Benjamini-Hochberg method in a , one-way ANOVA with Tukey’s post hoc test in b – d . Error bars, SEMs. Source data of a – d are provided as a source data file Full size image We next tested whether light-induced larval head cast was also regulated by the disinhibitory mechanism. We measured size of larval head cast in response to light-on using a light spot assay under a dim white light as larval head cast size saturated when light became perceivably high. We used relatively higher (26.34 pW/mm 2 , measured at 470 nm, see Methods) or lower (1.80 pW/mm 2 , measured at 470 nm) light intensity to elevate or lower the level of head cast size in controls, so as to make enough room for further decrease or increase in experimental groups. We first knocked down expression of GRD in the LRIN R13B07 s to mitigate the inhibition of LRIN R13B07 s by light. As shown in Fig. 4b , size of larval head cast upon light-on was significantly reduced in the GRD knockdown group as compared to that of the controls, at light intensity of 26.34 pW/mm 2 . This suggests that inhibition of the inhibitory LRIN R13B07 s was indeed necessary for larval aversive response to light. On the other hand at relatively weaker light intensity of 1.80 pW/mm 2 , when GAD or vGAT was downregulated in LRIN R13B07 s to reduce the GABAergic inhibitory input to CLPN R82B09 s, size of light-on-induced larval head casts was significantly enhanced (Fig. 4c ). In addition, knocking down RDL expression in CLPN R82B09 s to relieve the inhibition on CLPN R82B09 s also significantly enhanced size of larval head cast upon light-on at light intensity of 1.80 pW/mm 2 (Fig. 4d ). These results were consistent with our previous conclusion that disinhibtion of CLPN R82B09 s through inhibiting LRIN R13B07 s gated CLPN R82B09 s’ response to light since CLPN R82B09 s’ firing probability is positively related to the ratio of light-induced head cast over spontaneous head cast. As sizes of the light-induced head casts are usually larger than that of the spontaneous ones, CLPN R82B09 s’ firing probability is positively related to the measured head cast size. Next, to exclude the possibility that the increased head cast sizes resulted from the manipulations of neuronal activities even in absence of light, we performed the light spot assay with light constantly kept off, i.e. the light spot was actually dark. The differences in larval head cast in response to “light-on” were no longer observed (Supplementary Fig. 9a, b ). Thus, the increased head cast sizes were indeed the outcomes of the interaction between the neuronal activities and light stimulation. Taken together, larval head cast response to light-on was indeed facilitated by disinhibition of CLPN R82B09 s via LRIN R13B07 s. Re-inhibition on CLPN R82B09 s represses larval head cast Because light inhibition on LRIN R13B07 s was removed after the light was turned off (Fig. 1f ), we speculated that the inhibition of LRIN R13B07 s on CLPN R82B09 s would be naturally restored once the larva had exited the light spot. Further head cast would therefore be inhibited. 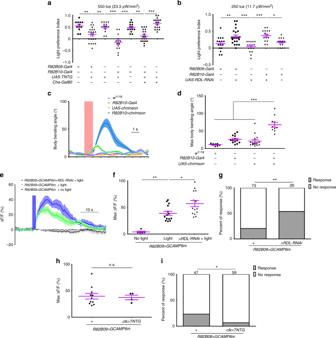Fig. 3 The CLPNR82B09s control head cast response to light.aInhibiting CLPNR82B09s abolishes larval avoidance to white light at 550 lux (23.3 μW/mm2).bKnocking down RDL expression in CLPNR82B09s enhances larval avoidance to white light at 250 lux (11.7 μW/mm2).c–dOptogenetic stimulation of CLPNR82B09s evokes larval head cast.dis the statistics of head cast sizes inc. The pink bar indicates the period of optogenetic stimulation.e–gKnocking down RDL expression in CLPNR82B09s increases both amplitude and probability of CLPNR82B09s’ response to light in calcium imaging. The blue bar ineindicates 470 nm light stimulation at intensity of 10.58 μW/mm2.fis the statistics of peak responses ine.h–iBlockingclk-LexAneurons with TNTG does not affect the amplitude (h), but undermines the probability of CLPNR82B09s’ response to light in calcium imaging (i). One second 470 nm light stimulation at intensity of 10.58 μW/mm2was used. Ine–i,R82B09>GCAMP6mis the short forUAS-GCAMP6m/+;R82B09-Gal4/+.R82B09>GCAMP6m+RDL-RNAiis the short forUAS-GCAMP6m/UAS-RDL-RNAi;R82B09-Gal4/+.clk>TNTG;R82B09>GCAMP6mis the short forclk-LexA/UAS-GCAMP6m; R82B09-Gal4/LexAop-TNTG. Numbers above columns ingandiindicate sample sizes. n.s. not significant, *P< 0.05, **P< 0.01, ***P< 0.001, one-way ANOVA with Tukey’s post hoc test ina–b,d, andf,t-test inh, fisher’s exact test ingandi. Error bars, SEMs. Source data ofa–iare provided as a source data file We then examined the role of LRIN R13B07 s-CLPN R82B09 s inhibition in head cast for larvae that had just exited the light spot. As expected, at relatively high light intensity of 26.34 pW/mm 2 , knocking down the light receiving receptor GRD in LRIN R13B07 s did not affect larval head cast size upon light exit as the absence of GRD did not affect LRIN R13B07 s-CLPN R82B09 s inhibition in darkness (Fig. 5a ). However, knocking down GAD or vGAT expression in the LRIN R13B07 s could significantly improve size of head cast upon light exit (Fig. 5b ), as could also be seen in the larvae with RDL downregulated in the CLPN R82B09 s (Fig. 5c ), at light intensity of 1.80 pW/mm 2 . The enhancement in larval head cast upon “light exit” was not seen if light was constantly kept off during the assay (Supplementary Fig. 9c, d ). These results meant that the stimulatory effect of light on larval head cast could persist even after light went off. The immediate restoration of the inhibition on CLPN R82B09 s prevented further head cast upon light exit. Fig. 5 Larval reorientation at light-off is repressed by reinhibition of CLPN R82B09 s. a – c Size of larval head cast at light-off in the light spot assay is unaffected by downregulation of GRD in LRIN R13B07 s ( a ), but is enhanced by down regulation of GAD/vGAT in LRIN R13B07 s ( b) or RDL in CLPN R82B09 s ( c) . d – e Knocking down GAD expression in LRIN R13B07 s ( d ) or RDL in CLPN R82B09 s ( e ) increases the rate of larva returning to light after light exit. Number above the columns indicates the sample sizes. f A cartoon showing the hypothesized working mechanism of the disinhibitory pathway in larval light avoidance. The large light blue circles indicate light spots. The circles with arrows are red for LRIN R13B07 , green for CLPN R82B09 , dark blue for clk-LexA labeled neurons and orange for unspecified excitatory neurons upstream of CLPN R82B09 s, respectively. Arrow heads indicate excitatory input. Bar heads indicate inhibitory input. The thickness of arrows indicates the strength of the inhibitory or excitatory effects. Light intensity in spot measured at 470 nm was 26.34 pW/mm 2 for a, 1.80 pW/mm 2 for b – e . n.s. not significant, * P < 0.05, ** P < 0.01, *** P < 0.001, one-way ANOVA with Tukey’s post hoc test in a – c , χ 2 -test with subgroup comparisons controlled by Benjamini-Hochberg method in d and e . Error bars, SEMs. Source data of a – e are provided as a source data file Full size image As head cast could potentially bring the larva back into the light spot after it had left, the immediate restoration of the LRIN R13B07 s-CLPN R82B09 s inhibition might help to secure the “correct” choice of light escape by repressing the potential larval head cast. We then tested this assumption by examining the chance for the larva to return to light spot after the initial light escape. Knocking down GAD expression in LRIN R13B07 s to prevent restoration of LRIN R13B07 s-CLPN R82B09 s inhibition indeed significantly increased the rate of larvae returning to light spot from no more than 15.00 to 39.02% (Fig. 5d , Supplementary Fig. 10 ). Similarly, knocking down RDL in the CLPN R82B09 s also increased the rate from 8.33 to 26.67% (Fig. 5e ). Thus, the restoration of inhibition on CLPN R82B09 s could help improve larval light avoidance by repressing potential improper head cast after the initial light escape. In this work, we discovered a disinhibitory neural mechanism that gated Drosophila larval head cast in presence and absence of light (Fig. 5f ). LRIN R13B07 s that exert a tonic inhibition on the larval head cast controlling CLPN R82B09 s are inhibited by light to facilitate the head cast response. Once the larva escapes from light successfully, the inhibition on CLPN R82B09 s is naturally restored to prevent further improper head casts, thus securing the success of light avoidance. Such a disinhibitory mechanism has several roles. First, the inhibition on CLPN R82B09 s represses larval behavioral response to light. This justifies the reduced larval responsiveness to very dim light that is usually safe. It also helps larvae to terminate behavioral response to light when necessary. Second, the inhibition of LRIN R13B07 s by light ensures the specificity of larval orientation in response to light, as the inhibition on CLPN R82B09 s prevents their excitation by non-visual stimulus. This specificity can be further enhanced if there exists another pathway for light to stimulate CLPN R82B09 s [34] . Third, the opposite regulation of reorientation at transitions between light and darkness enhances larval preference for darkness over light. In addition to the explicit light avoidance facilitated by the head cast upon light stimulation, light avoidance is also enhanced by the inhibition of further potential head casts after light escape, in an implicit manner. Compared with the recently reconstructed larval visual system that includes the first to third order neurons [13] , LRIN R13B07 s and CLPN R82B09 s should be at least the 3 rd or higher order neurons. For the known reconstructed second order visual neurons that likely project to region of LRIN R13B07 s’ dendrites, all are cholinergic except for pdf neurons [13] . As pdf neurons carry only part of the inhibitory signal to LRIN R13B07 s, those cholinergic neurons must activate some downstream inhibitory neurons that inhibit LRIN R13B07 s. pdf neurons themselves may also inhibit LRIN R13B07 s through other downstream neurons. Besides the second order neurons, one pair of third order glutamatergic visual projection local neurons also project to the region of LRIN R13B07 s’ dendrites. They may channel part of the inhibition on LRIN R13B07 s. As for CLPN R82B09 s, they are disinhibited by light through the disinhibitory pathway. As they are also susceptible to cholinergic excitatory input (Fig. 2j, k ), it is possible that CLPN R82B09 s can also be activated by light through cholinergic neurons. On the output side, as parts of dendritic termini of CLPN R82B09 s end in SEZ (Fig. 2d ), a region that has been suggested to be crucial for motor control [15] , [16] , [35] , CLPN R82B09 s may thus target onto the turning command neurons in SEZ to regulate larval head cast. It is likely that CLPN R82B09 s also control larval head cast response to aversive sensory stimulus in other modalities, such as gustation or olfaction. The observation that pdf neurons channel part of the light inhibition on LRIN R13B07 s prompts us to reconsider the role of pdf neurons in larval light avoidance. It has been well established that light could entrain larval clock and induce photophobic behaviors through Bolwig’s organs. Downstream to Bolwig’s organs, pdf neurons were known to mediate the entraining of clock, but their roles in light avoidance has been on debate [7] , [12] . Based on our observation, pdf neurons do have the potential to affect larval light avoidance through mediating the light inhibition on LRIN R13B07 s, although ablating pdf neurons did not significantly change CLPN R82B09 ’s response to light. It is possible that their role in light avoidance cannot be readily detected, unless light signal goes through those non-pdf neurons is lessened. One important property of LRIN R13B07 s in the disinhibitory neural circuit is that it is sensitive to dim light, although the light inhibition does not saturate even at high light intensities. But at behavioral level, the size of the disinhibition regulated larval head cast in response to dark-to-light transition seemed to saturate at moderate light intensity. Therefore, when larvae choose a dark or dim condition over a brighter condition, the light avoidance must involve the LRIN R13B07 s-CLPN R82B09 s disinhibitory circuit. For example, for feeding larvae that digs deep into food, the contrast between the light outside and the dark inside may provide part of the driving force as the opaque food surrounding larval eyes makes an almost completely dark local environment. On the other hand, when larvae choose between bright and brighter light, larval head cast in both conditions may saturate so that light avoidance may not happen. If it does, the disinhibition of CPLNs should not be involved. The disinhibitory control of light elicited larval turning behavior resembles the disinhibitory mechanism in vertebrates for motor program selection. In vertebrate, striatal neurons from motor cortex send inhibitory signal to inhibit pallidum neurons that exert tonic inhibition on spinal motor command neurons [20] . One advantage of this mechanism is the strict and precise control of motor initiation and termination. The adoption of disinhibitory mechanism in Drosophila larval motor control suggests that the higher level control of motor initiation is conserved among invertebrate and vertebrate. As most innate preferences are realized though reorientation, we suggest disinhibition to be a common neural mechanism underlying animal innate preference behavior. Fly culture and strains All flies were raised at 25 °C on standard medium and 12 h:12 h light/dark cycles of culture [36] . The following fly strains were used in this work: w 1118 , Rh5-eGFP(BL8600); Rh6-eGFP(BL7461), Rh6-Gal4(BL7464), GMR-myrRFP(BL7121), R13B07-Gal4(BL48545), R82B10-Gal4(BL46717), R82B09-Gal4(BL40133), R82B09-LexA(BL61613), clk-LexA(R43D05-LexA,BL54147), pdf-LexA [37] , Cha-Gal80, vGlut-Gal80, tsh-Gal80 [38] , GMR-Gal80, UAS-TNTG [39] , UAS-NaChBac [40] , UAS-GCAMP6m(BL42748) [41] , UAS-mCD8-GFP(BL5137), UAS-myrGFP(BL7118), UAS-Chrimson(BL55135) [42] , UAS-NpHR(BL41753) [43] , UAS-sytGFP,UAS-Denmark(BL33064) [44] , UAS-mCD8-RFP(BL32218), UAS-myrGFP,QUAS-mtdTomato(3xHA)(X); trans-Tango (II) [30] , hsFLP, UAS-FRT-rCD2-FRT-mCD8GFP, UAS-FRT-stop-FRT-Chrimson, UAS-FRT-stop-FRT-sytGFP, UAS-GAD-RNAi(TH02214.N), UAS-vGAT-RNAi(THU4304), UAS-RDL-RNAi(TH02821.N), UAS-GRD-RNAi(THU3884), LexAop-myrGFP(BL32209), LexAop-TNTG, LexAop-GCAMP6s(BL44273) [41] , LexAop-CD4::GFP 11 ;UAS-CD4::GFP 1-10 [37] , [45] , pdf-DTI [37] . The RNAi lines were from Qinghua Drosophila Stock center. Light/dark choice assay for larval light preference The protocol for test of larval light/dark preference was as previously reported [37] . In brief, 20 cleaned 3 rd instar larvae were placed on a 1.5% agar plate with one half covered with a taped lid. White light generated from a fluorescent light was placed above the plate to illuminate the uncovered half. Light intensity of 550 lux corresponded to 23.3 μW/mm 2 , 250 lux corresponded to 11.7 μW/mm 2 at maximal readings (S401C, Thorlabs, Inc). After 2 min of adaptation on agar plate, larvae were aligned along the light/dark boundary and allowed to move freely for 10 min. Then the numbers of larvae in each half of agar plate were scored. Experimental temperature was at 25.5 °C. Larval light preference index (PI) was calculated as: PI = (number of larvae in the dark half–number of larvae in the light half)/(number of larvae in the dark half + number of larvae in the light half). PIs were shown as mean ± SEM. Light spot assay The procedure of light spot assay was largely same as previously described [46] . Individual larva was first acclimated on an agar plate for 2 min in a dark room. The plate was rotated to re-orientate larva heading toward a light spot of 2 cm-in-diameter generated by a white light LED before start of test. The white light had one intensity peak at 450 nm with half width of 10 nm and another peak at 583 nm with half width of 65 nm. 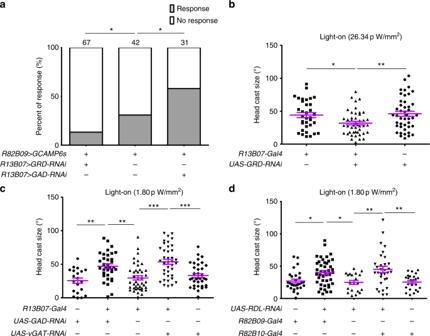Fig. 4 Larval reorientation at light-on is facilitated by disinhibition of CLPNR82B09s.aKnocking down GRD and GAD expression in LRINR13B07s, respectively, reduces and increases the probability for CLPNR82B09s to respond to light in calcium imaging. One second 470 nm light stimulation at intensity of 1.058 μW/mm2was used. Numbers above columns indicate sample sizes. Genotypes of larvae used areR82B09-LexA/UAS-GRD-RNAi;LexAop-GCAMP6s/R13B07-Gal4,R82B09-LexA/+;LexAop-GCAMP6s/+andR82B09-LexA/UAS-GAD-RNAi;LexAop-GCAMP6s/R13B07-Gal4, respectively.b–dSize of larval head cast at light-on in the light spot assay is reduced by downregulation of GRD in LRINR13B07s (b), but is enhanced by down regulation of GAD/vGAT in LRINR13B07s (c)or RDL in CLPNR82B09s (d). Light intensity in spot measured at 470 nm was 26.34 pW/mm2forb, 1.80 pW/mm2forc–d. *P< 0.05, **P< 0.01, ***P< 0.001,χ2-test with subgroup comparisons controlled by Benjamini-Hochberg method ina, one-way ANOVA with Tukey’s post hoc test inb–d. Error bars, SEMs. Source data ofa–dare provided as a source data file 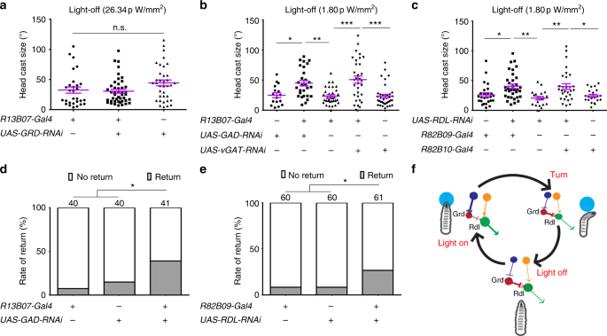Fig. 5 Larval reorientation at light-off is repressed by reinhibition of CLPNR82B09s.a–cSize of larval head cast at light-off in the light spot assay is unaffected by downregulation of GRD in LRINR13B07s (a), but is enhanced by down regulation of GAD/vGAT in LRINR13B07s (b)or RDL in CLPNR82B09s (c).d–eKnocking down GAD expression in LRINR13B07s (d) or RDL in CLPNR82B09s (e) increases the rate of larva returning to light after light exit. Number above the columns indicates the sample sizes.fA cartoon showing the hypothesized working mechanism of the disinhibitory pathway in larval light avoidance. The large light blue circles indicate light spots. The circles with arrows are red for LRINR13B07, green for CLPNR82B09, dark blue forclk-LexAlabeled neurons and orange for unspecified excitatory neurons upstream of CLPNR82B09s, respectively. Arrow heads indicate excitatory input. Bar heads indicate inhibitory input. The thickness of arrows indicates the strength of the inhibitory or excitatory effects. Light intensity in spot measured at 470 nm was 26.34 pW/mm2fora,1.80 pW/mm2forb–e. n.s. not significant, *P< 0.05, **P< 0.01, ***P< 0.001, one-way ANOVA with Tukey’s post hoc test ina–c,χ2-test with subgroup comparisons controlled by Benjamini-Hochberg method indande. Error bars, SEMs. Source data ofa–eare provided as a source data file The light intensity of 1.80 pW/mm 2 or 26.34 pW/mm 2 measured at 470 nm (S120C, Thorlabs, Inc.) in light spot was used. The whole process from larval entering to exiting of the light spot was video recorded with an infrared high-resolution web camera from above. The lens was covered by an 850 nm infrared narrow-pass filter to prevent the disturbance of visible light on video. Three 850 nm LED lights that were evenly placed around the plate to illuminate the arena. Experimental temperature was kept as 25.5 °C. Videos were analyzed with the software SOS and custom scripts (see below for larval head cast analysis). For larval re-entry to light spot, a larva that had its head touched the light spot for at least once within 20 s after the initial exit was defines as a larva of returning. Optogenetics Eggs of proper genotypes were laid on food supplied with 0.2 mM trans-retinal. For testing behavioral consequence of optogenetic activation of CLPN R82B09 s with Chrimson, cleaned single 3 rd instar larva was allowed to crawl on a 1.5% agar plate. A 620 nm red-light pulse was delivered onto the larva in periods of straight forward locomotion. The process of larval locomotion was video recorded and processed with SOS software and custom scripts (see below for larval head cast analysis). For imaging CLPN R82B09 ’s response to optogenetic inhibition of LRIN R13B07 s using NpHR, 540 nm green light was used (also see below for calcium imaging). Pharmacology Larval brain samples were prepared following previously reported protocols but with modifications [47] . Individual 3 rd instar larva was removed from food and washed alternatively with ddH 2 O and 70% ethanol for 1 min. It was dissected in standard saline solution (128 mM NaCl, 2 mM KCl, 4 mM MgCl 2 ⊡ 6H 2 O, 1.8 mM CaCl 2 , 36 mM sucrose, 5 mM HEPES, pH = 7.1) and the brain were transferred to 1.5 ml microcentrifuge tube with 500 μl standard saline containing 0.4 mg/ml protease (Sigma-Aldrich, P5147) and 0.1 mg/ml collagenase (Sigma-Aldrich, C0130). The brain was digested for ~3 h before being centrifuged at 1 rcf for 2.5 min. The digest solution was pipetted off and 100 μl Schnerder’s Drosophila Medium (Gibco, 21720–024) containing 10% FBS (Sera Pro, S601S-500) was added. Single brain was transferred into round shaped recording chamber (16 mm in diameter) filled with 1.5 ml standard saline for calcium imaging. To prevent the sample from moving during circulating, brain tissue was covered by a custom made stainless steel grids (mesh size 200, hole size 100 μm). During calcium imaging, drugs were added into the recording chamber using a circulating pump (LongerPump, BT100–2J). Drugs used included picrotoxin (Hellobio, HB0506), etomidate (Mechem Express, HY-B0100), GABA (Sigma-Aldrich, A5835) and acetylcholine chloride (Sigma-Aldrich,P6625). Calcium imaging Calcium imaging was similar to previous report [36] . Individual clean 3 rd instar larva was briefly dissected in AHL (Adult Hemolymph-Like) solution to expose central brain, but with the anterior part of body intact. It was then transferred with AHL solution into a chamber formed by reinforcing rings on a glass slide and covered with a cover slip. The target neuron was directly localized under two-photon microscope. For calcium imaging response to light stimulation, 470 nm blue light (470 nm at peak with half-width of 10 nm) of various intensities measured at 470 nm was used for both LRIN R13B07 s and CLPN R82B09 s. For calcium imaging response of CLPN R82B09 s to optogenetic inhibition of LRIN R13B07 s using NpHR, 540 nm green light was used. All Ca 2+ imaging experiments with light stimulation were performed with an Olympus FV-1000 two-photon microscope with ×40 water immersion lens. Infrared laser at 910 nm was used for excitation of GCAMP. The change in fluorescent intensity in neurons was captured by two-photon scanning at frequency of 2.33 frames per second and resolution of 256 × 256. For calcium imaging response of CLPN R82B09 s to drugs, experiments were performed with an Olympus FV-1000 confocal microscope with ×10 lens. Change in fluorescent intensity was captured at frequency of 1.75 frames per second and resolution of 320 × 320. For quantitative analysis of Ca 2+ imaging data, ImageJ (https://imagej.nih.gov/ij/) was used to batch process images to determine fluorescence intensity of regions of interest, i.e. the cell bodies of neurons. Average fluorescence intensity (F) in 20 sequential images before stimulation or drug application was used as the basal level. Changes in fluorescence intensity ( Δ F) were calculated and Δ F/F was used to indicate Ca 2+ responses. Specifically when measuring CLPN R82B09 s’ response to light, only responses of more than 20% increase in fluorescent intensity were considered as valid to overcome the possible effect of spontaneous oscillation. Immunochemistry and confocal microscopy Third instar larval brains were dissected from larvae in PBS, fixed in PBS containing 4% paraformaldehyde for 1 h at room temperature and washed 4 × 30 min in PBS containing 0.5% Triton X-100 (PBT) before being blocked for 2 h in PBT containing 5% goat serum. The samples were then incubated with primary antibodies (rabbit anti-GABA, 1:50, Cat. A2052, Sigma-Aldrich; rabbit anti-RFP 1:100, Cat. ab62341, Abcam; mouse anti-rCD2, 1:1000, Cat. 201305, Biolegend; rabbit anti-CD4, 1:200, Cat. ab133616, Abcam; mouse anti-PDF, 1:100, PDF-C7 concentrate, DSHB; mouse anti-Fas II, 1:100, 1D4 concentrate, DSHB; mouse anti-ChAT, 1:100, ChAT4B1 concentrate, DSHB; rat anti-HA, 1:200, Cat. 11867423001, Roche) overnight at 4 °C, before being washes in PBT for 4 × 30 min. Specifically, as QUAS-mtdTomato(3xHA) was the designed reporter for trans-Tango signal, we used anti-HA to visualize the trans-Tango signal. The samples were then incubated with secondary antibody (Alexa 647-conjugated goat anti-rabbit, 1:100, Cat. A27040, Alexa 647-conjugated goat anti-mouse, 1:100, Cat. A21235, Alexa 647-conjugated goat anti-rat, 1:100, Cat. A21247, or Dylight 594-conjugated goat anti-rat, 1:100, Cat. SA5–10020, all from Thermo Fisher) for 2 h at room temperature and washed in PBT 3 × 10 min in darkness before being mounted and viewed. Images were acquired using an Olympus FV-1000 confocal laser scanning microscope and subsequently processed with ImageJ (www.nih.gov/ij). Specifically for processing the images about GRASP between LRIN R13B07 s and CLPN R82B09 s, the GRASP signal was confirmed by continuously tracing the anti-CD4 signals that marked the morphology of LRIN R13B07 and CLPN R82B09 , so that they were separated from the non-specific GFP signals. Larval head cast analysis The larval behavioral details in light spot assay were analyzed with a modified version of SOS [46] . In brief, single larva was sketched out from background and thinned to a line by algorithms implanted in matlab (Mathworks Inc.). The two ends of the line, head, and tail, together with midpoint of the line and centroid obtained from the larval body outline, were used to calculate headspeed, tailspeed, midspeed, and cmspeed. The bending angle of larval body, headtheta, was calculated from the angle between head-midpoint line and midpoint-tail line. The angular speed of headtheta is termed headomega. For larval head cast size upon light-on and light-off in light spot assay, the size of head cast upon light-on was defined as previously described with modifications [46] . As larva head cast happened always after deceleration, they were considered as an assembly when we judged the light related events. First, periods in tailspeed was defined according to the fluctuation of tailspeed during larval peristalsis. Deceleration was defined if the minimum tailspeed in one period was lower than in the previous period for more than 15% and the maximum tailspeed was no higher than in the previous period. Multiple continuous deceleration periods joined into one deceleration segment. Second, the time window for picking the deceleration related head cast was defined in either of the following ways: if larval tailspeed dropped to a level below arbitrarily set threshold, the time window was the whole-subthreshold period; if the larval tailspeed after deceleration was above the threshold, the time window was from 1 tailspeed period before to 2 tailspeed periods after the end of the deceleration. Third, the largest head cast size in the time window that began within 2 tailspeed periods before or 4 tailspeed periods after larva entered light spot was picked as the size of head cast upon light-on. For head cast size upon light-off, the largest head cast size in the time window of 0.5–5 s after larva exit the light spot, or in the time window from 0.5 s after light exit to the re-entry of light if the re-entry was within 5 s after light exit, was picked as the size of head cast upon light off. The extracted values of head cast sizes were confirmed by reviewing the videos. Head cast data that didnot match with the videos due to improper image processing were discarded. Size of larval head cast in response to optogenetic stimulation of CLPN R82B09 s was extracted in a similar way as in response to light-on in light spot assay, except that a 5 s time window for measuring head cast size was set as from the beginning to 4 s after the ending of the 1 s red light stimulation The codes are available at http://www.github.com/zfgong/zpp . Statistics Statistics was performed with prism6.0 (Graphpad Inc.). Fisher’s exact test was used for comparing the rate of event occurrence between two groups. For comparing of event occurrence rate among three groups, we made use of the rcompanion package of R (version 3.5.0) and did χ 2 -test. The p -values between subgroup comparisons were adjusted using FDR (false discovery rate) controlled by the Benjamini-Hochberg method. For all the rest, t -test or one-way ANOVA with Tukey’s post hoc test were used. Error bars in scatter plot and shaded areas flanking curves represented SEM. The details of the statistics for relevant figure panels are in Supplementary Summary of Statistics.